Vibrational near-field mapping of planar and buried three-dimensional plasmonic nanostructures Nanoantennas confine electromagnetic fields at visible and infrared wavelengths to volumes of only a few cubic nanometres. Assessing their near-field distribution offers fundamental insight into light–matter coupling and is of special interest for applications such as radiation engineering, attomolar sensing and nonlinear optics. Most experimental approaches to measure near-fields employ either diffraction-limited far-field methods or intricate near-field scanning techniques. Here, using diffraction-unlimited far-field spectroscopy in the infrared, we directly map the intensity of the electric field close to plasmonic nanoantennas. We place a patch of probe molecules with 10 nm accuracy at different locations in the near-field of a resonant antenna and extract the molecular vibrational excitation. We map the field intensity along a dipole antenna and gap-type antennas. Moreover, this method is able to assess the near-field intensity of complex buried plasmonic structures. We demonstrate this by measuring for the first time the near-field intensity of a three-dimensional plasmonic electromagnetically induced transparency structure. Optical antennas in the visible as well as in the infrared and terahertz (THz) spectral region confine light to a deep subwavelength volume and can increase the light–matter interaction on the nanoscale [1] , [2] , [3] , [4] , [5] . Moreover, resonantly excited antennas show high local near-field intensities in the close vicinity of the antennas [6] , [7] , and thus make them suitable for sensing applications. In particular, antennas in the infrared region are of great interest as the molecular fingerprints are situated in this spectral domain. This enables vibrational spectroscopy to identify and detect extremely small quantities of molecular substances, which is of importance to industry, analytical science and medicine, for example, for early disease diagnosis or trace gas detection. Tailoring localized surface plasmons is the key for technologies based on surface-enhanced scattering [8] such as surface-enhanced Raman scattering [9] , [10] , [11] , [12] and surface-enhanced infrared spectroscopy [13] , [14] , [15] , [16] , [17] in which the sensitivity can be increased by several orders of magnitude. The core of these techniques is the control of resonances in plasmonic metallic nanoantennas, which exhibit enhanced near-field intensity. In the case of surface-enhanced infrared spectroscopy, the molecular vibrational absorption scales with the intensity of the field at the location of the molecule [18] and leads to an absorption feature in the far-field scattering spectrum. It is of crucial importance to assess the local near-field intensity of resonant antenna structures in the infrared region in order to optimize the coupling of the plasmon oscillation with the vibrational oscillation of the nearby molecules [19] , and hence enhance the vibrational signal in detection. Several techniques were employed in the past to map plasmonic near-fields. One of them is two-photon luminescence microscopy that is limited by optical diffraction [20] , [21] . This limit was overcome by using techniques such as electron energy loss spectroscopy [22] , [23] , cathodoluminescence [24] , [25] and photoemission electron microscopy [26] , [27] . These methods are mostly restricted to the visible or near-infrared region and would require high-resolution setups for the infrared region, being only sensitive to the surface. Also, for electron energy loss spectroscopy the samples need to be prepared on ultrathin membranes so that transmission electron microscopy (TEM) technology can work. In contrast, scanning near-field optical microscopy (SNOM) has been routinely used to map plasmonic near-fields in the visible as well as in the infrared spectral region [28] , [29] , [30] , [31] . However, mapping the near-fields of complex three-dimensional (3D) embedded antenna structures or plasmonic cavities [32] , [33] , [34] remains very challenging for electron energy loss spectroscopy, photoemission electron microscopy and cathodoluminescence. This is particularly true for SNOM, where mapping deeply below the surface is impossible due to the necessity of direct tip–sample interaction. Another technique for plasmonic near-field mapping is local refractive index sensing, which was used to derive the local near-field intensity [35] , [36] . In addition, photosensitive molecular probes around plasmonic structures were exposed via the plasmonic near-field intensity and subsequently imaged with scanning electron microscopy or atomic force microscopy [37] , [38] . Here, we present a new approach that uses the strength of a molecular vibration to directly map the near-field intensity of plasmonic nanostructures with a probe volume that is 1.4 × 10 −5 times the volume of the free space wavelength cubed. We measure the transmittance spectra of the antennas in the far-field with conventional Fourier transform infrared spectroscopy (FTIR) and extract the antenna-enhanced molecular vibrational strength of a molecular patch, as shown in Fig. 1 . The vibrational strength scales directly with the overlap of the local molecular probe with the local plasmonic near-field intensity. Like SNOM, our technique is suited for the infrared or THz spectral region. The unique advantage that makes our method an important complementary tool is its ability to incorporate the molecular probe into complex 3D buried antenna structures and measure their near-field intensities. For the first time we demonstrate experimentally the field distribution of a stacked and embedded plasmonic electromagnetically induced transparency (EIT) structure for the different plasmonic modes, which would not be possible with other state-of-the-art methods. 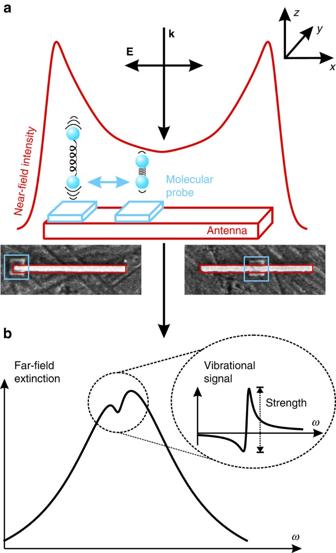Figure 1: Far-field antenna-enhanced spectroscopy mapping the plasmonic near-fields. (a) The gold antenna (red bar) is resonant to an incident far-field polarized along the long-axis of the antenna. The molecular patches (blue square) localized at different positions with respect to the gold nanoantenna serve as molecular probes of the local plasmonic near-field intensity. Vibrational modes are excited via the local near-field, where the oscillation strength depends on the near-field intensity. The scanning electron micrographs depict two different positions of the HSQ patches with respect to the antenna (length 1,400 nm). (b) The far-field extinction is measured by Fourier transform infrared spectroscopy. After baseline correction the vibrational signal is extracted to show a Fano lineshape, which stems from the coupling between the plasmon oscillation and the molecular vibration. The vibrational strength is defined as the difference between the maximum and the minimum of the vibrational signal. Figure 1: Far-field antenna-enhanced spectroscopy mapping the plasmonic near-fields. ( a ) The gold antenna (red bar) is resonant to an incident far-field polarized along the long-axis of the antenna. The molecular patches (blue square) localized at different positions with respect to the gold nanoantenna serve as molecular probes of the local plasmonic near-field intensity. Vibrational modes are excited via the local near-field, where the oscillation strength depends on the near-field intensity. The scanning electron micrographs depict two different positions of the HSQ patches with respect to the antenna (length 1,400 nm). ( b ) The far-field extinction is measured by Fourier transform infrared spectroscopy. After baseline correction the vibrational signal is extracted to show a Fano lineshape, which stems from the coupling between the plasmon oscillation and the molecular vibration. The vibrational strength is defined as the difference between the maximum and the minimum of the vibrational signal. Full size image Antenna-enhanced vibrational signal from localized molecules Using electron-beam lithography we fabricated 100 × 100 μm 2 large arrays of gold rod antennas as plasmonic structures. In a second electron-beam step, we positioned with an accuracy of 10 nm hydrogen silsesquioxane (HSQ) patches (200 × 200 × 30 nm 3 ) at defined locations with respect to the antennas, as shown in the scanning electron micrographs in Fig. 1a (see Methods for further information). The vibrational Si–H band at 2,252 cm −1 that is still present after patterning serves as the quantitative probe for our local near-field intensity (see Supplementary Fig. S1 ). 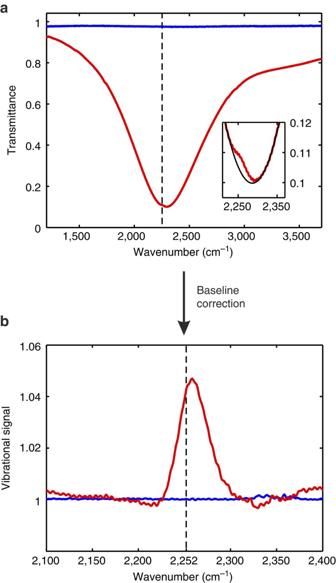Figure 2: Measured antenna-enhanced vibrational signal of nanoscopic HSQ patches. (a) The plot shows the measured transmittance of the antenna array with the HSQ patches positioned at one end of the antennas (as shown in the left micrograph inFig. 1a). The blue curve corresponds to incident light polarized perpendicular to the antenna axis (ypolarization). The red curve corresponds to incident light polarized along the long-axis of the antenna (xpolarization). In the plasmon resonance dip an absorption feature at 2,252 cm−1(black dashed line) from the Si–H vibration in the HSQ patch is observed. The inset zooms in at the vibrational feature in the plasmon dip. The black line is the lineshape of the plasmon resonance. (b) The vibrational signal of the HSQ patch after baseline correction is shown forxpolarization (red curve) andypolarization (blue curve). A pronounced absorption feature at 2,252 cm−1(black dashed line) is observed for excitation withx-polarized light where the plasmonic near-field intensity is resonantly enhanced, whereas no such feature is observed for excitation withy-polarized light. Figure 2a shows the measured transmittance of an antenna array, where we defined HSQ patches at only one end of the antenna as shown in the left scanning electron micrograph of Fig. 1a . When the polarization is set along the long-axis of the antenna ( x polarization, red curve) the transmittance exhibits a broad dip, due to the plasmon resonance of the gold nanoantenna next to the HSQ vibration. In the inset, this vibrational signature is observed on top of the plasmon resonance. The plasmon oscillation in the antenna is not excited when the polarization is set perpendicular to the antenna ( y polarization, blue curve), resulting in a flat transmittance spectrum. In order to extract the vibrational strength we conduct a baseline correction of the transmittance spectrum, namely dividing the transmittance spectrum of the antenna with the patch by the lineshape of the plasmon resonance. The vibrational strength is defined as the difference between the maximum and the minimum of the vibrational signal around 2,252 cm −1 , as schematically shown in Fig. 1b . In Fig. 2b we plot the vibrational signal for both polarizations. A vibrational feature is clearly observed for the resonant x polarization (red curve) and is absent for the off-resonant y polarization (blue curve) proving that our far-field vibrational signal solely stems from the plasmonically enhanced near-field intensity. The signal exhibits a Fano lineshape due to the interference of the spectrally broad plasmon oscillation with the spectrally narrow molecular vibration [39] , [40] , [41] . Figure 2: Measured antenna-enhanced vibrational signal of nanoscopic HSQ patches. ( a ) The plot shows the measured transmittance of the antenna array with the HSQ patches positioned at one end of the antennas (as shown in the left micrograph in Fig. 1a ). The blue curve corresponds to incident light polarized perpendicular to the antenna axis ( y polarization). The red curve corresponds to incident light polarized along the long-axis of the antenna ( x polarization). In the plasmon resonance dip an absorption feature at 2,252 cm −1 (black dashed line) from the Si–H vibration in the HSQ patch is observed. The inset zooms in at the vibrational feature in the plasmon dip. The black line is the lineshape of the plasmon resonance. ( b ) The vibrational signal of the HSQ patch after baseline correction is shown for x polarization (red curve) and y polarization (blue curve). A pronounced absorption feature at 2,252 cm −1 (black dashed line) is observed for excitation with x -polarized light where the plasmonic near-field intensity is resonantly enhanced, whereas no such feature is observed for excitation with y -polarized light. Full size image Spectroscopy of a nanoscopic molecular probe To map plasmonic near-fields we use the HSQ patches as local molecular probes and subsequently position them at different locations with respect to the antennas. As shown in the schematic of Fig. 3a we define the shift s as the distance from the left antenna end to the centre of the HSQ patch, taking negative values when the patch centre is outside the antenna. In the four scanning electron micrographs we show four fabricated patch positions where we shift the patch from the outside of the antenna ( s= −75 nm and s= −65 nm) to its left end ( s =+25 nm) and further to the centre of the antenna. In order to account for the detuning of the plasmon resonance due to the change in the local dielectric environment, we fabricated five different antenna lengths ranging from 1,400 nm to 1,600 nm with a 50-nm-step for each patch position. 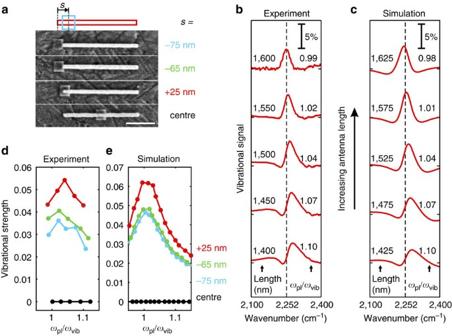Figure 3: Tuning the plasmonic antennas and shifting the molecular probe. (a) The scanning electron micrographs depict four different patch positionssof the HSQ patches with respect to the left end of the plasmonic antennas as shown in the schematic on top (scale bar 500 nm). (b) The vibrational signal is measured with the patch position fixed ats=+25 nm and the antenna length tuned from 1,400 to 1,600 nm with a 50 nm step. The detuningωpl/ωvibscales accordingly from 1.10 to 0.99. (c) Simulation results are in good agreement with experimental results. The spectral position of the vibrational band of HSQ at 2,252 cm−1is indicated by the black dashed lines and the spectra are vertically shifted. (d) The experimental vibrational strength as a function of the detuningωpl/ωvibis extracted for the four different patch positions,s=−75 nm (blue),s=−65 nm (green),s=+25 nm (red) and centre (black), as shown ina. For each patch position antennas with five different lengths were fabricated. (e) The vibrational strengths for more antenna lengths were extracted from numerical simulations. Figure 3b shows the measured vibrational signals with a fixed patch position s =+25 nm and the five different antenna lengths increasing from bottom to top spectrum. We define the detuning of the antenna plasmon resonance ω pl with respect to the vibrational resonance ω vib as the ratio ω pl / ω vib . The detuning demonstrates that the bottom spectrum stems from the coupling of a blue detuned plasmon oscillator with respect to the vibrational resonance, whereas the top spectrum stems from a slightly red detuned plasmon oscillator. Changing the length of the antennas, and hence the detuning of the plasmon resonance with respect to the vibrational band also changes the resonant lineshape due to Fano asymmetry (see Supplementary Fig. S2 ). Figure 3: Tuning the plasmonic antennas and shifting the molecular probe. ( a ) The scanning electron micrographs depict four different patch positions s of the HSQ patches with respect to the left end of the plasmonic antennas as shown in the schematic on top (scale bar 500 nm). ( b ) The vibrational signal is measured with the patch position fixed at s =+25 nm and the antenna length tuned from 1,400 to 1,600 nm with a 50 nm step. The detuning ω pl / ω vib scales accordingly from 1.10 to 0.99. ( c ) Simulation results are in good agreement with experimental results. The spectral position of the vibrational band of HSQ at 2,252 cm −1 is indicated by the black dashed lines and the spectra are vertically shifted. ( d ) The experimental vibrational strength as a function of the detuning ω pl / ω vib is extracted for the four different patch positions, s =−75 nm (blue), s =−65 nm (green), s =+25 nm (red) and centre (black), as shown in a . For each patch position antennas with five different lengths were fabricated. ( e ) The vibrational strengths for more antenna lengths were extracted from numerical simulations. Full size image We compare our experimental results to numerical simulations (see Fig. 3c , and see Methods and Supplementary Fig. S1 for further details). The numerical transmittance spectra are also baseline corrected to obtain the vibrational signal. The simulated antenna lengths are chosen in such a way that the detuning values ω pl / ω vib (indicated by labels on the right in the simulated spectra) match to the experimental detuning values. Very good agreement is obtained between the measured and simulated vibrational strength as well as the measured and simulated lineshape of the vibrational signal. To quantify the antenna-enhanced molecular vibration, we now plot the vibrational strength as defined in Fig. 1b for the different antenna lengths as a function of the detuning ω pl / ω vib and compare the experiment ( Fig. 3d , five antenna lengths) with the simulation ( Fig. 3e , 15 antenna lengths). The red curves correspond to the patch position s= +25 nm and depict the vibrational strengths extracted from the vibrational signals in Fig. 3b,c . The highest vibrational strength is observed when the molecular resonance and the antenna plasmon resonance overlap, which is also where we have the largest near-field intensity. Shifting the molecular patch away from the position s= +25 nm decreases the vibrational strength for all antenna lengths. The blue and green curves correspond to s= −75 nm and s= −65 nm, respectively. Strikingly, even a shift of only 10 nm reveals different vibrational strengths so that this small step size can be resolved experimentally. For the patch positioned at the centre of the antenna, the vibrational strength decreases substantially and is hard to detect (black curves). Direct mapping of near-field intensity of plasmonic antennas In addition to the four patch positions investigated in Fig. 3 , we fabricated five further patch positions to map directly the near-field intensity along the whole rod antenna. 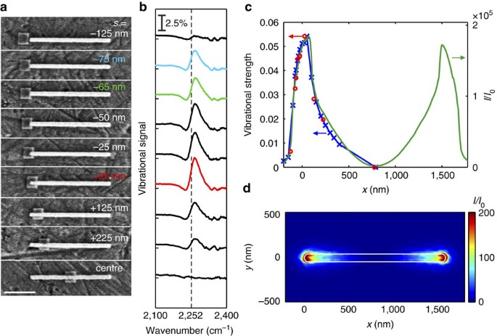Figure 4: Direct mapping of the near-field intensity of a dipole antenna. (a) The scanning electron micrographs show nine samples with different HSQ patch positions and a fixed antenna length (scale bar, 500 nm). (b) Measured vibrational signals for the nine samples (spectra shifted vertically) with the black dashed line indicating the vibrational band of HSQ at 2,252 cm−1. The scanning electron micrographs with coloured labels and the coloured spectra correspond to the patch positions ofFig. 3. (c) The red circles are the strength of the measured vibrational signal inbas a function of the patch position. The blue curve is the simulated vibrational strength for 19 different patch positions normalized to the experiment (multiplied by a factor 0.85). The green curve is the simulated near-field intensity enhancementI/I0summed up in the volume of the HSQ patch shifted in 10 nm steps along thexaxis.IandI0are the near-field intensities with and without antenna, respectively (I=|Ex|2+|Ey|2+|Ez|2). (d) The numerical calculated top view ofI/I0in the plane 10 nm above the antenna is shown for the dipole antenna. Figure 4a shows the scanning electron micrographs of the nine fabricated samples where we label the patch position s . The images with colour-coded labels are the patch positions corresponding to those investigated in Fig. 3 . In Fig. 4b we plot the vibrational signals for a fixed antenna length of 1,500 nm for the different patch positions that are shifted vertically for clarity, corresponding to the scanning electron micrographs in Fig. 4a . By fabricating five different antenna lengths for each of the nine patch positions (see Supplementary Fig. S3 ), we can pick the antenna length that is in resonance with the vibrational band. We observe a continuous increase in the vibrational signal starting from the patch at the centre to the patch at the left end ( s =+25 nm, red curve). Shifting the patch further to the outside of the antenna decreases the vibrational signal again. Figure 4: Direct mapping of the near-field intensity of a dipole antenna. ( a ) The scanning electron micrographs show nine samples with different HSQ patch positions and a fixed antenna length (scale bar, 500 nm). ( b ) Measured vibrational signals for the nine samples (spectra shifted vertically) with the black dashed line indicating the vibrational band of HSQ at 2,252 cm −1 . The scanning electron micrographs with coloured labels and the coloured spectra correspond to the patch positions of Fig. 3 . ( c ) The red circles are the strength of the measured vibrational signal in b as a function of the patch position. The blue curve is the simulated vibrational strength for 19 different patch positions normalized to the experiment (multiplied by a factor 0.85). The green curve is the simulated near-field intensity enhancement I/I 0 summed up in the volume of the HSQ patch shifted in 10 nm steps along the x axis. I and I 0 are the near-field intensities with and without antenna, respectively ( I=|E x | 2 +|E y | 2 +|E z | 2 ). ( d ) The numerical calculated top view of I/I 0 in the plane 10 nm above the antenna is shown for the dipole antenna. Full size image In Fig. 4c we plot the dependence of the vibrational strength as a function of patch position. The red circles are extracted from Fig. 4b . The blue curve is composed of simulations for 19 patch positions for the resonant antenna length, where we normalize the curve to the maximum vibrational strength in experiment. A steep peak is observed around the end of the antenna in the experiment as well as in the simulation. We specifically find that the vibrational strength is 8.4 (±0.9) times higher for the patch at the left end of the antenna ( s =+25 nm) than for the patch outside the antenna ( s =−125 nm). The green curve is the ratio of the near-field intensity I along the x axis of the resonant antenna and the near-field intensity I 0 with no antenna present. By shifting the probe volume in 10 nm steps and integrating the near-field intensity enhancement in the volume the green curve is obtained. A very good agreement between the vibrational signals probed in the far-field as a function of the patch position (red circles and blue curve) and the near-field intensity (green curve) is obtained. From this we infer that our method is very sensitive not only to lateral field distributions ( Fig. 4d ) but also to the field distribution in the z direction, generally depending on the probe volume. We attribute the small differences for x >0 nm (inside the antenna) to modified volumes of the patch in the experiment when it is in contact with the antenna. The lateral resolution is determined by the lateral dimensions of the molecular patch (200 × 200 nm 2 ). It can be improved by reducing the patch size, as will be discussed below. In SNOM experiments the near-field power dependence of the recorded signal varies with the relative strengths of the scattering channels that contribute dominantly to the far-field signal radiated by the object and the antenna [18] , [42] . Here, we observe a strictly linear dependence of our vibrational signal on the near-field intensity. From this we conclude that the scattering process into the far-field via the antenna is a negligible process in our experiment (see Supplementary Fig. S4 ). Moreover, due to the small size of the molecules, resonantly enhanced absorption by the vibrational transition is orders of magnitude larger than scattering. This result can be derived from ab intio calculations, and is also suggested by the typical cross-sections of a small dipole for scattering C scat a 6 / λ 4 and absorption C abs a 3 / λ (with a being its characteristic size) [43] . Here, the processes are resonant in the mid-infrared, which makes the scattering cross-section much smaller than in the visible or near-infrared. This confirms that our vibrational spectroscopy is well-suited for direct near-field mapping. An absolute enhancement factor of the signal strength can be estimated by comparing the plasmonically enhanced vibrational signals to non-enhanced vibrational signals of HSQ. Here we obtain factors of about 270. This number is significantly smaller than values reported in literature [16] , [44] . We attribute this to two effects: first, the hotspots located at the antenna ends are not completely covered with HSQ; second, the sampling is performed over the patch volume resulting in smaller signal enhancements. We now apply our method to plasmonic gap-type antennas. Scanning electron micrographs of the antennas are shown in Fig. 5a . We position HSQ patches at the gap (top image), at both ends (centre image) and at one end of the antennas (bottom image). We fabricated three different gap sizes (55 nm, 65 nm and 75 nm) and five different antenna lengths for each patch position and measured transmittance spectra (see Supplementary Fig. S5 for all vibrational strengths). We plot in Fig. 5b the vibrational signal for antennas with 55-nm gap. We observe a 5.9 (±0.2) times enhancement in the vibrational strength with the patch at the gap (pink curve) compared with the patch at the left end of the antenna (orange curve). As the near-field intensity distribution at the ends of the gap antenna is symmetric, the vibrational strength simply doubles when we place one patch at each end (green curve) instead of one patch at the left end (orange curve). The indicated detuning values ω pl / ω vib show that the gap-antennas are slightly red detuned from the molecular vibration. Hence, we would expect a slightly higher vibrational signal at the gap when we tune the antennas further to the blue due to the higher near-field intensity. 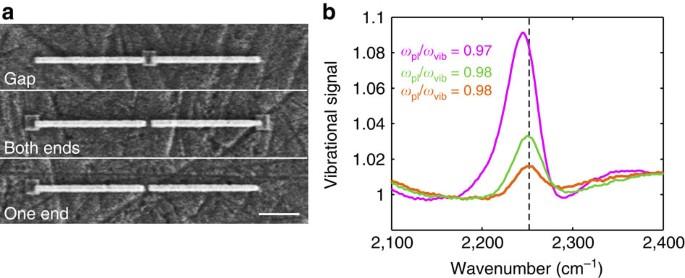Figure 5: Direct mapping of the near-field intensity for gap-type antennas. (a) Scanning electron micrographs of the gap-type antennas with the patch positioned at the gap, at both ends, and at one end are shown (scale bar, 500 nm). (b) Vibrational signals with the patch at the gap (pink curve), at both ends (green curve) and at one end (orange curve) are compared for a 55-nm gap size. The signal of the patch at the gap is enhanced 5.9 times compared with that of the patch at one end. The black dashed line indicates the vibrational band of HSQ at 2,252 cm−1. Figure 5: Direct mapping of the near-field intensity for gap-type antennas. ( a ) Scanning electron micrographs of the gap-type antennas with the patch positioned at the gap, at both ends, and at one end are shown (scale bar, 500 nm). ( b ) Vibrational signals with the patch at the gap (pink curve), at both ends (green curve) and at one end (orange curve) are compared for a 55-nm gap size. The signal of the patch at the gap is enhanced 5.9 times compared with that of the patch at one end. The black dashed line indicates the vibrational band of HSQ at 2,252 cm −1 . Full size image Near-field intensity of 3D plasmonic antennas Recently, it has been shown that SNOM is capable of mapping plasmonic near-fields of subsurface plasmonic scatterers [45] . Nevertheless, this technique relies on the interaction of the tip with the plasmonic near-field, which decays rapidly with increasing distance from the structure. Hence, resolution and depth contrast also decrease. The vibrational signal obtained with our method solely depends on the overlap of the molecular probe with the plasmonic near-field intensity. Therefore, it is perfectly suitable for assessing the near-field intensity of deeply buried 3D antenna structures via incorporating the molecular probe at specific positions into the antenna structure. With this, we measure the near-field intensity at the edge of the bright and the dark resonator of a stacked plasmonic EIT-structure for the different modes [34] . 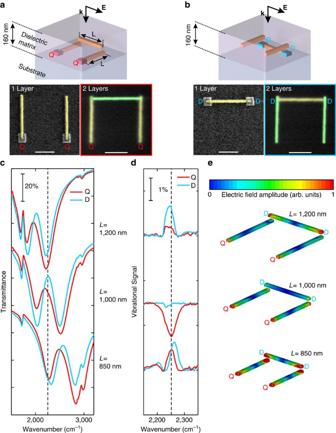Figure 6: Measured plasmonic near-field of a 3D buried plasmonic EIT-structure. (a,b) Schematic view and scanning electron micrographs (patches not visible in the dielectric matrix; scale bars, 500 nm) of the two-layer EIT-structure embedded in a 160-nm thick dielectric matrix (PC403). Q (red) and D (blue) indicate the patch positions at the quadrupole and the dipole, respectively. (c) Transmittance spectra for increasing structure size (spectra shifted vertically) with the lower-energy bright mode, the dark mode and the higher energy bright mode tuned to the HSQ vibration, respectively. The spectral position of the HSQ vibration is indicated by the black dashed line. Red (blue) curve is the transmittance when the patches are positioned at the quadrupole (dipole). (d) Vibrational signals for the three different modes with patches at the quadrupole (red curves) and dipole (blue curves), which are supported by the simulated electric field amplitude on the structure surface in (e). Figure 6a (Fig. 6b ) shows a schematic of the structure and scanning electron micrographs where we positioned two patches near the quadrupole (dipole) and stacked a dipole (quadrupole) on top of it. The quadrupole is the double wire and the dipole is the single one. The thickness of the spacer layer is 100 nm and we spin-coated an additional 60 nm capping layer on top. Due to the near-field coupling of the dipole (bright resonator) and the quadrupole (dark resonator), a low-energy and high-energy bright mode can be observed in the transmittance spectra with a transparency window in between (dark mode). This is shown in Fig. 6c where we increased the length L of the dipole and quadrupole rods from the bottom to the top spectrum to tune the three modes to the HSQ vibration at 2,252 cm −1 , indicated by the black dashed line. The red curves depict the measured transmittance with the molecular patches at the quadrupole as probe for the quadrupolar near-field and the blue curves show the measured transmittance with the molecular patches at the dipole as probe for the dipolar near-field. The absorptive features around 1,740 and 2,900 cm −1 stem from vibrational excitations in the dielectric matrix PC403. In Fig. 6d the vibrational signals at 2,252 cm −1 are extracted. Considering the vibrational signals corresponding to the low-energy bright mode (bottom spectrum) we observe a clear signal from the dipolar near-field (blue curve) as well as from the quadrupolar near-field (red curve) where the signal is slightly lower. For the dark mode (middle spectrum) a clear signal is observed for the quadrupole (red curve), which is not present for the dipole (blue curve). For the second bright mode at higher frequencies (top spectrum) a higher signal for the dipole is again observed when compared with the quadrupole. These experimental observations are in very good agreement with the near-field simulations shown in Fig. 6e . At the dark mode (centre antenna structure), mostly the quadrupole is excited and nearly no charge oscillation occurs in the dipole; hence the quadrupole exhibits stronger near-fields. For the bright modes (top and bottom structures) strong near-fields at the dipole and the quadrupole are observed where the dipole fields exhibit quantitatively higher field strengths. Figure 6: Measured plasmonic near-field of a 3D buried plasmonic EIT-structure. ( a , b ) Schematic view and scanning electron micrographs (patches not visible in the dielectric matrix; scale bars, 500 nm) of the two-layer EIT-structure embedded in a 160-nm thick dielectric matrix (PC403). Q (red) and D (blue) indicate the patch positions at the quadrupole and the dipole, respectively. ( c ) Transmittance spectra for increasing structure size (spectra shifted vertically) with the lower-energy bright mode, the dark mode and the higher energy bright mode tuned to the HSQ vibration, respectively. The spectral position of the HSQ vibration is indicated by the black dashed line. Red (blue) curve is the transmittance when the patches are positioned at the quadrupole (dipole). ( d ) Vibrational signals for the three different modes with patches at the quadrupole (red curves) and dipole (blue curves), which are supported by the simulated electric field amplitude on the structure surface in ( e ). Full size image We have positioned nanoscopic molecular probes with 10 nm accuracy on top of infrared plasmonic planar nanoantennas as well as into 3D antenna structures deeply buried in a dielectric matrix. By measuring the transmittance and extracting the molecular vibrational strength, we have quantitatively and reproducibly mapped the near-field intensities of resonant dipole and gap antenna structures as well as of a 3D plasmonic EIT-structure. We found excellent agreement with numerical simulations. Our method is able to map plasmonic fields from the near-infrared to the THz spectral region, as a large amount of molecular vibrational fingerprints is available in this spectral region. The variety of linewidth, vibrational strength, and spectral location combined with the positioning accuracy of electron-beam lithography makes our technique an extremely versatile tool. The spectral resolution is determined by the linewidth of the molecular vibrational band. Compared with other molecular bands, for example, the bands around 1,100 cm −1 of HSQ (see Supplementary Fig. S1 ), we have used a rather weak vibrational mode. Choosing a strong vibrational absorption can increase the sensitivity of our method by orders of magnitude, and will enable the use of much smaller probe volumes to achieve higher spatial resolution and measure the near-field intensities of single antennas with high luminosity setups. Furthermore, we have shown that the incorporation of the molecular probes in layer-by-layer processed 3D buried nanostructures [33] , [34] is a straightforward task and enables, for the first time, the mapping of plasmonic near-fields in all three dimensions. It is important to mention that the signal of our technique is due to the coupling of vibrational IR-transitions in molecules and plasmonic resonances, leading to Fano lineshape in the spectrum. We investigate for the first time the interaction of a narrow-band vibrational oscillator and a broadband plasmonic oscillator in the infrared with sub-wavelength spatial resolution, both at resonance as well as when slightly detuned. This is very different to SNOM, where the tip has a spectrally rather flat response in the given frequency region. Our results give detailed insight into light–matter coupling with spatially and spectrally resolved interaction at the nanoscale. With this we were also able to prove that the plasmonically enhanced molecular vibration scales linearly with the local near-field intensity, and molecular absorption in the mid-IR is the dominant process. We believe that our technique will trigger important experiments of plasmonically enhanced light–matter coupling down to the single molecule level using 3D plasmonic antenna structures that enable optimal coupling efficiencies. A small modification of the presented approach is the formation of nanoscopic self-assembled monolayers [46] in predefined holes on top of plasmonic antennas instead of patterning molecular patches. The advantage is the well-defined orientation of the molecules with respect to the antenna surface [16] , [19] and could allow the mapping of the individual field-vector components [47] by controlling the orientation of the molecules. Additionally, mapping the optical density of states of plasmonic antenna structures or high-Q cavities in the visible and near-infrared spectral region has been carried out via decay pathways branching into radiative and non-radiative decay channels [25] , [48] , [49] . Our approach of incorporating molecular vibrational absorptions at well-defined locations can be extended in the future to spatially map the radiative channels via absorption pathways. This may lead to new possibilities of radiation engineering with plasmonic structures and cavities in the infrared and THz spectral region. Numerical calculations The CST-Microwave Studio was used to calculate the transmittance spectra and the near-field distributions. A Drude-model was applied to describe the dielectric function of gold with the plasma frequency ω plasma =1.37 × 10 16 rad s −1 and the collision frequency ω coll =1.4 × 10 14 rad s −1 . The CaF 2 substrate was implemented into the calculation domain with a refractive index n =1.4. To model the HSQ-material, a Lorentz-model was fitted to the measured extinction of a 30-nm continuous HSQ-film after it was patterned with electron-beam lithography (see Supplementary Fig. S1 ). The complex dielectric function was extracted from the fit. Sample fabrication Gold nanorods were fabricated on top of a CaF 2 substrate with electron-beam lithography. First, a layer of polymethyl methacrylate was spin-coated onto the substrate. The nanostructures as well as markers were defined with the electron-beam and the sample was developed afterwards. Thermal evaporation of a 50-nm-thick gold film with 2 nm Cr adhesion layer and a subsequent lift-off process were performed to obtain the metalized structures. In a second processing step a HSQ layer was spin-coated and the patches were exposed with electron-beam lithography [50] . The markers from the first processing step ensured correct alignment of the HSQ patches with respect to the gold nanoantennas. A two-layer stacking approach with a step in between to position the HSQ patches was used to fabricate the plasmonic EIT-structure. Again, preprocessed gold markers were used to obtain good alignment for the HSQ patches as well as for the second gold layer. After the first gold layer and the HSQ positioning step PC403 was spin-coated resulting in a 100-nm-thick spacer layer. The top gold layer was capped with another 60 nm layer of PC403. Fourier transform infrared spectroscopy measurements Transmittance spectra of the antenna arrays were obtained using a Fourier transform infrared spectrometer (Bruker Vertex 80) combined with an infrared microscope (Bruker Hyperion), which is equipped with a 15 × Cassegrain objective (numerical aperture NA=0.4) and a liquid N 2 -cooled mercury cadmium telluride detector. The polarization of the incident light is controlled by an infrared polarizer. The measured sample spectra were normalized with respect to a bare CaF 2 substrate as the background. The background and the subsequent sample spectrum were collected with a resolution of 2 cm −1 and 2,500 scans with a mirror repetition rate of 40 KHz. How to cite this article: Dregely, D. et al. Vibrational near-field mapping of planar and buried 3D plasmonic nanostructures. Nat. Commun. 4:2237 doi: 10.1038/ncomms3237 (2013).